Evidence for zoonotic potential of ovine scrapie prions Although Bovine Spongiform Encephalopathy (BSE) is the cause of variant Creutzfeldt Jakob disease (vCJD) in humans, the zoonotic potential of scrapie prions remains unknown. Mice genetically engineered to overexpress the human prion protein (tgHu) have emerged as highly relevant models for gauging the capacity of prions to transmit to humans. These models can propagate human prions without any apparent transmission barrier and have been used used to confirm the zoonotic ability of BSE. Here we show that a panel of sheep scrapie prions transmit to several tgHu mice models with an efficiency comparable to that of cattle BSE. The serial transmission of different scrapie isolates in these mice led to the propagation of prions that are phenotypically identical to those causing sporadic CJD (sCJD) in humans. These results demonstrate that scrapie prions have a zoonotic potential and raise new questions about the possible link between animal and human prions. Transmissible spongiform encephalopathies (TSE), or prion diseases, are fatal neurodegenerative disorders that affect a large spectrum of mammalian species. These conditions include for instance, scrapie in small ruminants, bovine spongiform encephalopathy (BSE) in cattle and chronic wasting disease (CWD) in wild cervids. In humans, the most common form of TSE is sporadic Creutzfeldt-Jakob disease (sCJD), which affects ~1–2 individuals per million of the population per year and is generally observed in people aged over 50 years. In the absence of identified external causes sCJD is considered to be a spontaneous disorder precipitated by mis-folding of the normal cellular prion protein (PrP C ) [1] . It has been known for several centuries that scrapie is endemic in small ruminant animals used for human food production [2] . Despite this dietary exposure, epidemiological studies have failed to identify any clear link between scrapie and TSE occurrence in humans [3] , [4] . This apparent lack of zoonotic transmission by scrapie is considered to be a consequence of the transmission barrier phenomenon that naturally limits the propagation of prions from one species to another [5] . In 1996, a new human prion disease, referred as variant CJD (vCJD), was observed in UK individuals. Several lines of evidence have indicated that vCJD is the probable consequence of dietary exposure of humans to the agent responsible for epizootic of bovine spongiform encephalopathy (BSE) in UK cattle [6] . The occurrence of vCJD has provided significant evidence to show that the transmission barrier does not constitute an absolute protection against the zoonotic risk of prions that circulate in animal populations. This suggests that the need for an in-depth assessment of the permeability of the human species barrier to animal TSE agents including those responsible for scrapie in sheep. The potential diversity of scrapie prions has been investigated over many years by serial transmission of field isolates to the natural host of this condition, inbred mouse lines or as more recently to bank voles and mice with transgenic expression of different PrP sequences [5] , [7] . On the basis of the transmission features in conventional mice (incubation periods, distribution of the lesions in the brain), early transmission experiments described a considerable diversity of the scrapie agents with up to 20 prion strains reportedly identified [8] . However, more recent strain typing in transgenic mouse lines that express ovine PrP has identified a more restricted range that comprises at least four phenotypically distinct scrapie strains [5] , [9] , [10] , [11] , [12] . Despite converging evidence that scrapie is caused by a variety of prion strains, there is at this stage no comprehensive description of their diversity. A fundamental event in prion propagation is the conversion of the normal cellular prion protein (PrP C , which is encoded by the PRNP gene) into an abnormal disease-associated isoform (PrP Sc ) in tissues of infected individuals. PrP C is completely degraded by digestion with proteinase K (PK), whereas PrP Sc is N terminally truncated resulting in a PK resistant core, termed PrP res (ref. 13 ). According to the prion concept, PrP Sc is the principal if not sole component of the prion agent [14] and PrP res is a disease marker for prion diseases [13] , [15] . Particular biochemical properties of PrP Sc , such as detergent solubility, PK resistance and electromobility in western blotting (WB) can be used to distinguish between different prion agents or strains [16] , [17] . After identification of the gene encoding PrP, it was soon discovered that differences in amino-acid sequence between host PrP C and donor PrP Sc were the main driver for the transmission barrier. For example, the resistance of wild-type mice to clinical disease induced by hamster scrapie is abrogated by transgenic expression of hamster PrP C in mice [18] , [19] . However, it is also established that strain properties have a significant impact on the ability of prions to cross the species barrier. This is evidenced by studies showing that human vCJD isolates can be transmitted readily to conventional mice but that it is extremely difficult for sCJD isolates to propagate in the same mouse lines [20] , [21] . Furthermore, the amino-acid sequence of PrP Sc influences the efficacy of interspecies prion transmissions as tgHu models indicate that the human species barrier is more permeable to sheep-passaged BSE compared with its cattle counterpart [22] . Conceptually, the permeability of the prion transmission barrier is considered to be driven at the molecular level by the conformational compatibility between host PrP C and the misfolded strain-specific protein assemblies of PrP Sc that are present within infectious prion particles [23] . As a consequence, mice genetically engineered to express human PrP (tgHu), in the absence of endogenous mouse PrP, have emerged as relevant animal models to assess prion transmission across the human species barrier [24] . A major determinant of the susceptibility to human prion disease is Met/Val dimorphism at codon 129 of the PRNP gene [25] , [26] , and tgHu mice lines exist that express these variants of human PrP [27] . These tgHu mouse lines propagate human prions without an apparent species barrier and have been successfully used to confirm the zoonotic ability of the BSE agent from cattle [6] , [22] , [28] . In addition, prion transmission studies in tgHu mouse lines have highlighted that L-type atypical BSE in cattle displays a higher capacity to cross the human species barrier than does classical BSE in cattle, the prion strain responsible for vCJD emergence [29] , [30] . In the context of the Met/Val dimorphism in human PrP C and the potential diversity of sheep scrapie strains, it is clear that assessment of the permeability of human species barrier to ovine prions presents a considerable challenge [8] , [31] . In this study, we inoculated tgHu mice transgenic for expression of human PrP codon 129 variants intracerebrally with a panel of (i) biologically distinct ovine scrapie isolates, (ii) human prions and (iii) cattle BSE prions. The serial transmission of different scrapie isolates in tgHu mice led to the propagation of prions that were phenotypically identical to those that cause sporadic CJD (sCJD) in humans. Scrapie isolates transmit in tgHu mice We initially performed serial transmission studies in three tgHu mouse lines. These mouse lines were homozygous for methionine (tg Met 129 / tg340) or valine (tgVal 129 /tg361) at codon 129 of human PrP, or were their F1 cross (methionine/valine heterozygotes at codon 129; tgMet/Val 129 ). All of these mouse lines expressed human PrP approximately fourfold more compared with that seen in normal human brain tissue ( Fig. 1 ). 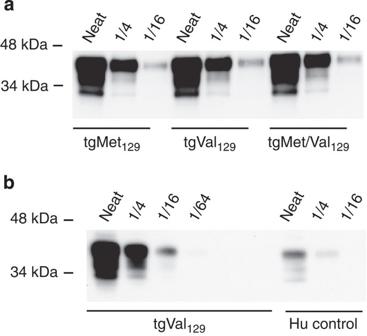Figure 1: PrPCexpression in tgHu mice. Brain homogenate dilutions (neat or 1/4, 1/8, 1/16 diluted in Laemmli’s buffer) were analysed by SDS–PAGE and western blot using 12% acrylamide gel. Normal PrP was detected using the monoclonal antibody 3F4 (0.8 μg ml−1). (a) tgMet129, tgMet/Val129and tgVal129samples. (b) tgVal129and human control brain samples. The three mouse lines were inoculated intracerebrally with a panel of six sheep scrapie isolates that had been collected between 1994 and 2002 from flocks naturally affected with this prion disease ( Table 1 ). The scrapie isolates were selected on the basis of the different transmission profiles they showed when inoculated in murine (tga20), bovine (tgBov/tg110) and ovine (tgShpXI and tg338) PrP transgenic mouse lines ( Fig. 2 ), which were indicative that they contained different ovine prion strains [5] , [27] . Figure 1: PrP C expression in tgHu mice. Brain homogenate dilutions (neat or 1/4, 1/8, 1/16 diluted in Laemmli’s buffer) were analysed by SDS–PAGE and western blot using 12% acrylamide gel. Normal PrP was detected using the monoclonal antibody 3F4 (0.8 μg ml −1 ). ( a ) tgMet 129 , tgMet/Val 129 and tgVal 129 samples. ( b ) tgVal 129 and human control brain samples. Full size image Table 1 Intracerebral inoculation of tgHu mice with a panel of human, bovine and ovine prion isolates. 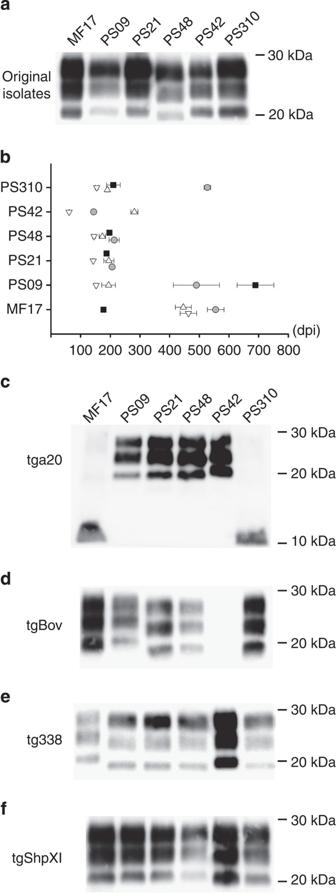Figure 2: Transmission properties of scrapie isolates in PrP transgenic mice. (a) The PrPreswestern blot pattern of six different natural sheep scrapie isolates (MF17, PS09, PS21, PS48, PS42 and PS310) was established using a monoclonal antibody Sha31. This panel of scrapie isolates was inoculated in transgenic mice (n=6 per group) that express the murine (tg20-grey circle), the bovine (tgBov-black square), the ovine A136R154Q171(tgshpXI-triangle up) and the ovine V136R154Q171(tg338-triangle down) PrP variants. For each isolate two serial passages were carried out: (b) the incubation period (mean±s.d.) as days post inoculation (dpi) of the second passage in the different mouse lines and (c–f) the PrPreswestern Blot profiles (10% brain homogenate) observed after two passages in each of the mouse lines. Full size table Figure 2: Transmission properties of scrapie isolates in PrP transgenic mice. ( a ) The PrP res western blot pattern of six different natural sheep scrapie isolates (MF17, PS09, PS21, PS48, PS42 and PS310) was established using a monoclonal antibody Sha31. This panel of scrapie isolates was inoculated in transgenic mice ( n =6 per group) that express the murine (tg20-grey circle), the bovine (tgBov-black square), the ovine A 136 R 154 Q 171 (tgshpXI-triangle up) and the ovine V 136 R 154 Q 171 (tg338-triangle down) PrP variants. For each isolate two serial passages were carried out: ( b ) the incubation period (mean±s.d.) as days post inoculation (dpi) of the second passage in the different mouse lines and ( c – f ) the PrP res western Blot profiles (10% brain homogenate) observed after two passages in each of the mouse lines. Full size image At completion of the first passage, none of the challenged tgHu mice developed clinical disease ( Table 1 ). However, western blot analysis showed weak but consistent disease-associated PK resistant PrP (PrP res ) accumulation in the brains of two tgMet/Val 129 mice inoculated with MF17 scrapie isolate ( Table 1 , Fig. 3a ). We considered the PrP res was not due to residual inoculum but rather to the conversion of tgHu PrP C into PrP Sc . Consequently, first passage mouse brains from each scrapie isolate transmission group were pooled and re-inoculated to the same tgHu line ( Table 1 ). Following second passage of sheep scrapie in the tgHu mouse lines clinical disease was observed in a proportion of the tgMet 129 and tgMet/Val 129 mice inoculated with four of the isolates ( Table 1 ). Western blot analysis confirmed the accumulation of PrP res in the brain of these second passage mice ( Fig. 3b ). There were no clinical signs of prion disease or PrP res accumulation observed in control mice inoculated with PBS or prion-free control brain homogenate, which had also undergone two serial passages ( Table 1 ). These controls confirmed that the prion disease observed in inoculated tgHu mice inoculated with the sheep scrapie isolates was not the consequence of a spontaneous PrP conversion and that cross-mouse contamination was unlikely. 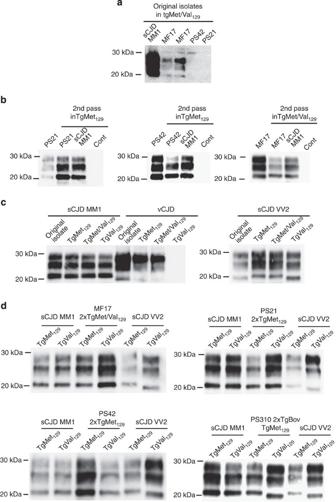Figure 3: PrPresdetection in scrapie-inoculated tgHu mice. TgMet129, tgVal129and their F1 cross tgMet/Val129mice were inoculated (n=6 per group) with (a) various natural sheep scrapie isolates (seeTable 1- MF17, PS21, PS42 and PS310); and (b) the same scrapie isolates after primary passage in tgHu mice. (c) The same mouse lines were challenged with MM1 and VV2 sporadic Creutzfeldt-Jakob disease (sCJD) and variant CJD (vCJD) isolates. (d) tgMet129and tgVal129mice were inoculated with scrapie isolates that had been previously passaged twice in human PrP (tgMet129or tgMet/Val129) or bovine PrP transgenic mice (tgBov, seeTables 3and4). PrPresdetection was carried out by SDS–PAGE and western blot with an anti-PrP monoclonal antibody Sha31. Figure 3: PrP res detection in scrapie-inoculated tgHu mice. TgMet 129 , tgVal 129 and their F1 cross tgMet/Val 129 mice were inoculated ( n =6 per group) with ( a ) various natural sheep scrapie isolates (see Table 1 - MF17, PS21, PS42 and PS310); and ( b ) the same scrapie isolates after primary passage in tgHu mice. ( c ) The same mouse lines were challenged with MM1 and VV2 sporadic Creutzfeldt-Jakob disease (sCJD) and variant CJD (vCJD) isolates. ( d ) tgMet 129 and tgVal 129 mice were inoculated with scrapie isolates that had been previously passaged twice in human PrP (tgMet 129 or tgMet/Val 129 ) or bovine PrP transgenic mice (tgBov, see Tables 3 and 4 ). PrP res detection was carried out by SDS–PAGE and western blot with an anti-PrP monoclonal antibody Sha31. Full size image Relative efficacy of scrapie and BSE transmission in tgHu To determine the susceptibility of tgHu mice to a prion strain with known zoonotic potential, we inoculated human PrP mouse lines with two different cattle BSE isolates. At first passage there was either an absence or an inefficient transmission of bovine prions in tgMet 129 and tgMet/Val 129 mice ( Table 1 ), although the attack rate significantly increased at second passage. No transmission or brain PrP res accumulation was observed in tgVal 129 mice inoculated with either of the two BSE isolates ( Table 1 ). These results concur with the commonly held view that a substantial species barrier limits the transmission of cattle BSE to humans [6] , [22] , [28] . The data also support the contention that the relative permeability of the human species barrier (as modelled here by the intracerebral transmission in tgHu mice) to cattle BSE and scrapie is not fundamentally different. Impact of scrapie adaptation in bovine PrP transgenic mice Sheep scrapie prions can be propagated experimentally in cattle and the hypothesis that BSE is derived from cattle exposure to scrapie remains a prominent theory [32] , [33] , [34] . Moreover, PrP Sc amino-acid sequence can strongly influence cross-species prion transmission [22] , [23] . In this context, the isolates that we obtained after two passages of sheep scrapie isolates in bovine PrP transgenic mice (tgBov) ( Fig. 2 ) were also inoculated into tgMet 129 tgHu mice ( Table 2 ). On the first passage, clinical signs were observed in a proportion of tgMet 129 mice inoculated with each of the tgBov-adapted sheep scrapie isolates. Similar transmission properties were also observed with scrapie isolate PS48 that failed to propagate in tgHu mice after two passages ( Table 1 ). These observations support the contention that the adaptation of ovine scrapie prions to the bovine PrP amino-acid sequence increases their capacity to propagate in tgHu mice. Table 2 Intracerebral inoculation of transgenic mice that express human PrP with ovine scrapie isolates previously adapted in bovine PrP transgenic mice. Full size table Lack of transmission barrier for human prions in tgHu mice In parallel to the inoculation with sheep scrapie isolates, we also inoculated the tgHu mice with human brain material from one vCJD and two sCJD patients. The sCJD cases were classified as Met/Met type 1 (MM1) and Val/Val type 2 (VV2), respectively [35] , based on the patient’s PRNP genotype at codon 129 and on the PrP res western blot profiles of these samples. On first passage, 100% of the tgHu mice inoculated with the two sCJD isolates developed clinical disease while the vCJD isolate was only propagated in tgMet 129 and tgMet/Val 129 mice ( Table 1 ). Differences in incubation periods ( Table 1 ) together with PrP res molecular profile and PrP res distribution patterns in the tgHu mouse brains concurred with the view that the vCJD, sCJD MM1 and sCJD VV2 isolates contained biologically distinct prions ( Figs 3c and 4 ). As expected, there was no reduction in incubation period during the second passage of sCJD and vCJD isolates in tgHu mice, which indicated the absence of a measurable species barrier between these human prions and the human PrP transgenic mice. 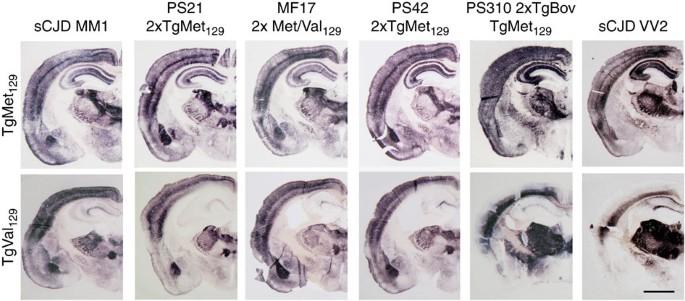Figure 4: Brain PrPresdeposition pattern in sCJD and scrapie inoculated tgHu mice. TgMet129or tgVal129mice were inoculated with MM1 and VV2 sCJD isolates. The same mouse lines were challenged with different natural sheep scrapie isolates (seeTable 1-MF17, PS21, PS42 and PS310) that had been serially transmitted (two passages) in tgMet129, tgMet/Val129(seeTable 1) or in mice that expressed bovine PrP (tgBov, seeTables 2and3). PK-resistant PrP detection was carried out by PET blot using an anti-PrP monoclonal antibody Sha31. Scale bar, 150 μm. Figure 4: Brain PrP res deposition pattern in sCJD and scrapie inoculated tgHu mice. TgMet 129 or tgVal 129 mice were inoculated with MM1 and VV2 sCJD isolates. The same mouse lines were challenged with different natural sheep scrapie isolates (see Table 1 -MF17, PS21, PS42 and PS310) that had been serially transmitted (two passages) in tgMet 129 , tgMet/Val 129 (see Table 1 ) or in mice that expressed bovine PrP (tgBov, see Tables 2 and 3 ). PK-resistant PrP detection was carried out by PET blot using an anti-PrP monoclonal antibody Sha31. Scale bar, 150 μm. Full size image Scrapie and sCJD display identical phenotypes in tgHu mice The molecular profile of disease-associated PrP that accumulated in scrapie inoculated PrP res -positive tgHu mice was distinct from that observed in the original sheep isolates. In contrast, the PrP res that accumulated in tgHu mice after inoculation with either sCJD or scrapie shared a similar molecular profile ( Fig. 3b ). These data suggested that transmission of sCJD and sheep scrapie prions in mice that expressed human PrP might have resulted in the propagation of same prion strain. To confirm this, brain homogenates prepared from clinical prion diseased tgHu mice inoculated with either sheep scrapie ( Table 3 ) or sheep scrapie adapted in tgBov ( Table 2 ) were re-passaged in tgMet 129 and tgVal 129 mouse lines. All the inoculated samples induced a 100% transmission attack rate in both tgHu mouse lines. The incubation periods ( Tables 2 and 3 ), together with the molecular profile ( Fig. 3d ) and distribution of PrP res ( Fig. 4 ) in the brains of these mice, were similar to those observed in similar animals inoculated with either VV2 or MM1 sCJD isolates. Strikingly, the transmission profiles of the majority of sheep scrapie prions in tgHu mice displayed a phenotype that was identical to MM1 sCJD. However, one of the sheep scrapie isolates that had been adapted in tgBov (PS310, Table 2 ) showed the same phenotype as the VV2 sCJD isolate ( Figs 3d and 4 ). Table 3 Intracerebral inoculation of tgHu mice with human sCJD cases and sheep scrapie isolates adapted (two passages) in tgMet 129 mice or tgMet/Val 129 . Full size table Similar results are obtained in a different tgHu mouse line To rule out the possibility that the phenomena we observed were a consequence of the particular tgHu mouse lines used, we inoculated a subset of the panel of bona fide sheep scrapie isolates into tg650 mice, which overexpress (approximately six fold) human PrP Met 129 (ref. 29 ). In a manner similar to that seen in the Met 129 tg340 mouse line, no clinical disease was observed on first passage of the sheep scrapie isolates in Met 129 tg650 mice ( Table 4 ). However, two tg650 mice (inoculated with two different scrapie isolates) were western blot-positive for PrP res in the brain. The second passage in tg650 mice of isolate PS21 (using brain homogenate prepared from a PrP res positive mouse on first passage) resulted in a 100% transmission attack rate. After third passage in tg650 mice, the incubation period of PS21 was 155±3 days, which was identical to MM1 sCJD in this mouse line [36] . The molecular profile and distribution of PrP res in the brain of tg650 mice inoculated with PS21 were identical to those observed in the same mouse line after inoculation with sCJD MM1 prions ( Fig. 5 ). Table 4 Intracerebral inoculation of tg650 transgenic mice with a panel of sheep scrapie isolates. 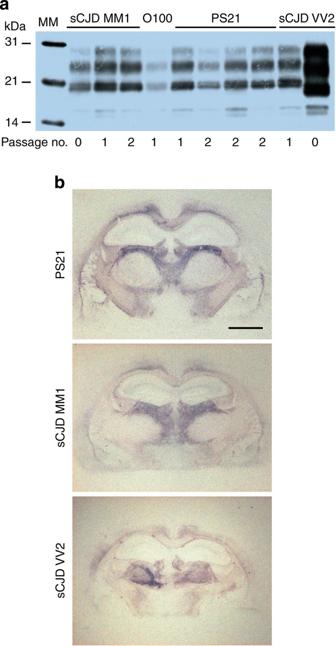Figure 5: PrPresin the brains of prion-inoculated tg650 transgenic mice. Transgenic mice (tgMet129/tg650) that overexpress the methionine variant at codon 129 of human PrP were inoculated with different natural sheep scrapie isolates (ov), cattle BSE (bov), human (hu) vCJD and sCJD samples (MM1 and VV2). Brains from first and/or second passage tg650 mice were tested for the presence of PrPresby (a) western blot (Sha31anti-PrP antibody) and (b) histo Blot (3F4 anti-PrP antibody). Scale bar, 160 μm. Full size table Figure 5: PrP res in the brains of prion-inoculated tg650 transgenic mice. Transgenic mice (tgMet129/tg650) that overexpress the methionine variant at codon 129 of human PrP were inoculated with different natural sheep scrapie isolates (ov), cattle BSE (bov), human (hu) vCJD and sCJD samples (MM1 and VV2). Brains from first and/or second passage tg650 mice were tested for the presence of PrP res by ( a ) western blot (Sha31anti-PrP antibody) and ( b ) histo Blot (3F4 anti-PrP antibody). Scale bar, 160 μm. Full size image Historically, non-human primate models were considered as the reference model for testing the permeability of the human species barrier with regards to prion transmission [37] , [38] . The successful transmission of cattle BSE prions to marmosets [39] and cynomolgus macaques [40] was considered as a strong argument in support of its zoonotic potential. While data related to the transmission of ovine scrapie in primates remain very limited, the intracerebral challenge of marmosets with one sheep scrapie isolate (PG 85/02) induced a typical prion disease with a shorter incubation time than that observed after challenge with cattle BSE [39] , suggesting an equivalent or higher ability of sheep scrapie to cross the species barrier. In contrast, other experiments failed to demonstrate the transmissibility of scrapie in non-human primates [41] . However, divergence exists between such these non-human primate and human PrP amino-acid sequences, which only show 96 to 99% homology. Furthermore, a number of experimental transmissions in PrP transgenic or wild-type animals indicate that one single amino-acid difference in the PrP sequence can markedly alter the issue of cross-species transmission [42] , [43] . In our view, these observations raise some concerns with regards to the relevance of primates as a model of human species barrier. The transmission experiments reported here unambiguously show that sheep scrapie prions propagate in mice that express variants of human PrP. While the efficiency of transmission at primary passage was low, subsequent passages resulted in a highly virulent prion disease in tgHu Met 129 and Val 129 mice. Transmission of different scrapie isolates in tgHu mice leads to the emergence of prion strain phenotypes that showed similar characteristics to those displayed by MM1 or VV2 sCJD prion isolates passaged in the same mouse lines. Change in phenotype is a common phenomenon associated with the transmission of prions across a species barrier [44] , [45] . Our observation that phenotypically similar prion strains emerged following transmission of different sheep scrapie isolates in tgHu mice is consistent with the concept that the range of PrP Sc conformations, which are considered to reflect prion strain diversity, is limited for a given PrP sequence. This restriction on PrP Sc conformations implies that prion propagation in hosts of a given PrP sequence results in a predefined range of prion strains [23] , [46] , [47] . An unexpected result of this study was the finding that transmission of sheep scrapie isolates in tgHu mice resulted in the emergence of prions with a similar phenotype to those associated with sCJD. As this result was obtained in two different tgHu mouse lines, we consider that our data support the view that passage of sheep scrapie prions across a human transmission barrier can lead to the emergence of sCJD prions. Other recent studies have similarly reported that, after one passage, no clinical disease or PrP res accumulation could be observed in tgHu mice overexpressing the human PrP following intracerebral challenge with a panel of scrapie isolates [48] . This observation concurs with our data here whereby propagation of sheep scrapie in tgHu mice was only clearly evident after second passage in these mouse lines. A similar phenomenon was also reported in a number of tgHu mouse models following the inoculation of cattle BSE [6] , [22] , [28] . This is a likely consequence of the strong transmission barrier limiting the propagation of both scrapie and BSE prions in mice that express human PrP. Our data were obtained by transmission studies in mice that overexpress human PrP and are in contrast with the reported lack of transmission of sheep scrapie isolates in human PrP knock-in mice [49] . However, while no species barrier is expected for transmission of human prions in tgHu mice, a significant proportion of sCJD isolates propagates with limited efficiency in human PrP knock-in mice [50] . This suggests that mice that express physiological levels of PrP might not be the most appropriate animal model to assess the permeability of the human species barrier to animal prions. Do our transmission results in tgHu imply that sheep scrapie is the cause of sCJD cases in humans? This question challenges well-established dogma that sCJD is a spontaneous disorder unrelated to animal prion disease. In our opinion, our data on their own do not unequivocally establish a causative link between natural exposure to sheep scrapie and the subsequent appearance of sCJD in humans. However, our studies clearly point out the need to re-consider this possibility. Clarification on this topic will be aided by informed and modern epidemiological studies to up-date previous analysis that was performed at the end of the last century [3] , [4] . The value of such an approach is highlighted by the implementation in the year 2000 of large-scale active animal TSE surveillance programs around the world that provided an informed epidemiological-based view of the occurrence and geographical spread of prion disease in small ruminant populations [51] . The fact that both Australia and New-Zealand, two countries that had been considered for more than 50 years as TSE-free territories, were finally identified positive for atypical scrapie in their sheep flocks provides an example of how prion dogma can be reversed [52] . However, the incubation period for prion disease in humans after exposure to prions via the peripheral route, such as in iatrogenic CJD transmission and Kuru, can exceed several decades [53] , [54] . In this context, it will be a challenge to combine epidemiological data collected contemporarily in animal populations and humans to investigate the existence of a causative link between prion disease occurrence in these different hosts. Furthermore, it is crucial to bear in mind that sporadic sCJD in humans is a rare disease (1–2 individuals per million of the population per year) and that scrapie has been circulating in small ruminants populations used for food purposes for centuries. Consequently, it is our opinion that even if a causative link was established between sheep scrapie exposure and the occurrence of certain sCJD cases, it would be wrong to consider small ruminant TSE agents as a new major threat for public health. Despite this, it remains clear that our data provide a new impetus to establish the true zoonotic potential of sheep scrapie prions. TSE isolates All the isolates used in this study were prepared as 10% (w/v) brain homogenates in 5% glucose. vCJD and sCJD isolates were obtained from the UK CJD reference centre in Edinburgh. The experimental protocol, including the use of human samples, was approved by the competent ethical committees (UK National CJD Research & Surveillance Unit Tissue bank: REC reference number 2000/4/157). All the sheep scrapie isolates, except one, were selected from the tissue archive of UMR INRA ENVT 1225. These scrapie isolates correspond to clinically suspect field cases that were collected between 1994 and 2004 from naturally affected commercial flocks in France. For each isolate, the exon 3 of the PrP encoding gene was sequenced [55] , [56] . All these sheep scrapie cases were confirmed positive by histopathology (identification of vacuolar changes in the brainstem). MF17 was a 5.5-year-old sheep, homozygous for ARQ at codons 136, 154 and 171 of the sheep PrP gene (ARQ/ARQ). PS09 was a 2.5-year-old ARQ/ARQ. PS21 was a 2.5-year-old ARQ/ARQ sheep. PS48 was a 5-year-old sheep, homozygous for VRQ at codons 136, 154 and 171 of the sheep PrP gene (VRQ/VRQ). PS42 was a 1.5-year-old VRQ/VRQ sheep. PS310 was a 7.5-year-old ARQ/ARQ sheep. The O100 scrapie isolate (inoculated in tg650 mice) was provided by the National French reference laboratory for scrapie diagnosis (ANSES, Lyon, France) and had been collected from a VRQ/VRQ sheep of unknown age. Transgenic mouse lines Transgenic mouse lines that express PrP C of different species were used to propagate the selected panel of TSE isolates: tgBov (or tg110, bovine PrP), tg338 (ovine V 136 R 154 Q 171 PrP), tgShXI (ovine A 136 R 154 Q 171 PrP variant). Except for the bovine PrP expressing mice (tg110) these mice lines were established on the same PrP null background mouse line (PrPKo) (Zurich I) [57] , [58] , [59] . The relative PrP expression level in the brain of these mouse lines in comparison with the natural host species was of the order: tg338, six- to eightfold; tg110, eightfold,; tgShpXI, three- to fourfold [27] . Tg340 and tg361 mouse lines that express human PrP methionine at codon 129 or valine at codon 129, respectively, in a PrPKo background, were generated following the same procedure as described for tg340 mice [22] . Both tg340 and tg361 are homozygous for human PRNP gene and tgMet/Val 129 mice used in our experiments were obtained by mating tg340 and tg361 mice (F1 generation). Mouse bioassays All animal experiments were performed in compliance with our institutional and French national guidelines in accordance with the European Community Council Directive 86/609/EEC. The experimental protocol was approved by the INRA Toulouse/ENVT ethics committee. Six- to ten-week-old female mice were anaesthetized and inoculated with 2 mg of brain equivalent (20 μl of a 10% brain homogenate) in the right parietal lobe using a 25-gauge disposable hypodermic needle. Mice were observed daily and their neurological status was assessed weekly. When clinically progressive TSE disease was evident, or at the end of their lifespan, animals were killed and their brains collected. Half of the isolated brain from those animals that had displayed TSE clinical signs was fixed by immersion in 10% formol and the other half was frozen at −20 °C. Tissues from found dead animals were frozen (no formalin fixation). Spleens from animals were not systematically collected (in particular in found dead animals) and data related to PrP Sc accumulation in this tissue are not available. Survival time was expressed as the mean of the survival days post inoculation (d.p.i.) of all the mice scored positive for PrP res , with its corresponding s.d. In cages where no clinical signs were observed, mice were killed at the end of their natural lifespan (650 to 800 days). In those cases, incubation periods reported in the table (>650 to 750 d.p.i.) corresponded to the survival time observed in at least three out of the six mice. Brain homogenates from PrP res positive mice, when available, were used for serial tranmission. When all mice were scored negative for PrP res on primary passage, PrP res -negative brain homogenates of animals that survived for more than 500 d.p.i. were used for the next passage. Anti-PrP monoclonal antibodies The anti-PrP monoclonal antibodies used in this study (kindly provided by J.Grassi, CEA, France) were Sha31 (epitope: 145 YEDRYYRE 152 ) and 3F4 anti-PrP (epitope: 111 HMAGAAAA 118 ) [60] . PrP res western blot detection Frozen brain tissue (175±20 mg) was homogenized in 5% glucose in distilled water in grinding tubes (Bio-Rad) adjusted to 10% (w/v) using a TeSeE TM Precess 48 homogenizer (Bio-Rad). A western blot kit (TeSeE WB kit Bio-rad) was used following the manufacturer’s recommendations and PrP res detection used a monoclonal antibody Sha31 at a dilution of 1/8,000. All the original western blot images are presented as Supplementary Data ( Supplementary Figs 1–12 ). Paraffin-embedded tissue blot and histoblot Paraffin-embedded tissue sections were collected on a 0.45-μm nitrocellulose membrane, before drying and deparaffinization. PK digestion (250 μg ml −1 , 2 h per 55 °C; Roche 1373200) was performed before denaturation into isothiocyanate guanidium solution (3 M, 10 min, at room temperature). Immunodetection was carried out with a monoclonal antibody Sha31 (4 μg ml −1 ) followed by an alkaline phosphatase coupled secondary antibody (Dako. Cat. No. D0314) at a dilution of 1/500). Alkaline phosphatase activity was revealed using NBT/BCIP substrate chromogen [61] . For the histoblotting procedure, brains ( n =3 per treatment group) were rapidly removed from killed mice and frozen on dry ice. Cryosections were cut at 8–10 mm, transferred onto Superfrost slides and kept at −20 °C until use. Sections were transferred to a nitrocellulose membrane (wetted in lysis buffer Nonidet P-40/0.5% sodium deoxycholate/100 mM NaCl/l0 mM EDTA/10 mM Tris-HCl, pH 7.8); the glass slides were quickly and immediately pressed onto the membrane for 25 s. Membranes were then submitted to PK (Roche ref 1373200) digestion (250 μg ml −1 , 2H, 55 °C) before denaturation into isothiocyanate guanidium solution (3M, 10 min, at room temperature). PrP res was probed using the anti-PrP monoclonal antibody 3F4 (concentration: 0.6 μg ml −1 ), followed by an alkaline phosphatase coupled secondary antibody (Dako ref D0314 at a dilution of 1/500). Enzymatic activity was revealed using NBT/BCIP substrate chromogen [29] . How to cite this article : Cassard, H. et al. Evidence for zoonotic potential of ovine scrapie prions. Nat. Commun. 5:5821 doi: 10.1038/ncomms6821 (2014).